Spatial-temporal model for silencing of the mitotic spindle assembly checkpoint The spindle assembly checkpoint arrests mitotic progression until each kinetochore secures a stable attachment to the spindle. Despite fluctuating noise, this checkpoint remains robust and remarkably sensitive to even a single unattached kinetochore among many attached kinetochores; moreover, the checkpoint is silenced only after the final kinetochore-spindle attachment. Experimental observations have shown that checkpoint components stream from attached kinetochores along microtubules towards spindle poles. Here we incorporate this streaming behaviour into a theoretical model that accounts for the robustness of checkpoint silencing. Poleward streams are integrated at spindle poles, but are diverted by any unattached kinetochore; consequently, accumulation of checkpoint components at spindle poles increases markedly only when every kinetochore is properly attached. This step change robustly triggers checkpoint silencing after, and only after, the final kinetochore-spindle attachment. Our model offers a conceptual framework that highlights the role of spatiotemporal regulation in mitotic spindle checkpoint signalling and fidelity of chromosome segregation. Mitosis is a key process of the eukaryotic cell cycle. Accuracy during mitosis ensures equal partitioning of chromosomes into two daughter cells [1] . Perturbation of mitosis can result in aneuploidy, an aberration in chromosome number, which is responsible for many diseases [2] , [3] . Fidelity of mitosis is the result of feedback controls [4] . Cyclin B is the ultimate determinant that drives mitotic progression; the cyclin B level must increase to drive nuclear envelope breakdown and formation of the bipolar microtubule spindle [4] , [5] . Cyclin B is also needed to establish proper chromosome-spindle attachment at each kinetochore (the outer centromere region of the chromosome [6] ). On chromosome congression, cyclin B must be degraded quickly via the anaphase-promoting complex/cyclosome (APC/C) to initiate the irreversible processes of anaphase onset and chromosome segregation [4] . While cyclin B controls mitotic progression, kinetochore-spindle attachments dictate the timing of cyclin B degradation [7] . Due to the dynamic nature of microtubules, initial attachments between microtubules and a kinetochore may be incorrect [1] . A powerful surveillance mechanism—called the mitotic spindle assembly checkpoint (SAC)—is activated at any aberrantly attached or unattached kinetochore [1] . The active SAC signal is generated only from mis/unattached kinetochores, and SAC activation requires cyclin B [8] , [9] , [10] . Active SAC signals propagate throughout the entire cytoplasm [11] , [12] , [13] , [14] , [15] , [16] , [17] , [18] , [19] , [20] to inhibit APC/C activation and cyclin B degradation. Only after all chromosomes are properly attached and congressed by the spindle, does SAC become inactivated to allow APC/C activation, cyclin B degradation and anaphase onset [1] . This checkpoint surveillance mechanism is highly sensitive and efficient. A single unattached chromosome can delay anaphase onset for hours, even while all other chromosomes (>20) have established stable spindle attachments [21] , [22] . Previous models attribute the high sensitivity of SAC signalling to a biochemical bistable switch that arises from mutual inhibition between cyclin B, SAC proteins and APC/C [23] . Specifically, cyclin B promotes SAC activity, which in turn inhibits APC/C, and active APC/C degrades cyclin B and inhibits SAC. Kinetochore attachments serve as input signals; the last kinetochore attachment toggles the switch, and drives irreversible silencing of SAC and degradation of cyclin B. However, recent findings indicate that reversible and irreversible SAC-silencing processes coexist [24] . For most of metaphase, perturbation of any kinetochore-spindle attachment reverses SAC silencing and APC/C activation; APC/C only becomes irreversibly activated immediately (<5 min) before anaphase onset. This intriguing observation indicates that additional factors, not yet incorporated into existing models, are important for irreversible SAC silencing. More importantly, schemes of SAC silencing that primarily focus on kinetochores have problems regarding robustness. A single unattached kinetochore does not constitute a robust input signal in these schemes. Suppose a cell has 20 kinetochores and each contributes 5% of the total SAC activity, given 10–30% protein-level fluctuations in cellular conditions [25] (for example, ≥10% for SAC proteins [26] ), it would be difficult for that cell to distinguish the last kinetochore-spindle attachment from the penultimate attachment via a signal increase of just 5%. Consequently, such a cell may enter anaphase prematurely before each kinetochore is properly attached. Yet, experiments demonstrated extremely high precision of anaphase onset, which occurs only after the last kinetochore-spindle attachment becomes stable [21] . Therefore, a biochemical bistable switch that solely depends on kinetochore attachments as input signals is insufficient for determining proper timing of SAC silencing. Furthermore, no existing model accounts for the spatiotemporal patterns of SAC activity [23] , [27] , [28] , [29] . This patterned activity may well have important biological functions. SAC proteins are highly colocalized with the bipolar spindle. They originally accumulate on unattached kinetochores [30] , [31] , [32] , [33] , [34] , but on stabilization of a proper kinetochore-spindle attachment, they undergo dynein-mediated poleward streaming along the spindles towards the associated spindle pole [11] , [35] , [36] , [37] , [38] . Furthermore, such poleward streaming is continuous until anaphase onset [37] , [39] , [40] . Inhibiting the poleward streaming causes mitotic arrest [35] , [36] , [41] , [42] . In addition, cyclin B degradation reportedly initiates from the spindle poles [43] , [44] , [45] , [46] , [47] . From these observations, three key questions arise. Why does cyclin B degradation start at spindle poles given that SAC inactivation is believed to occur at kinetochores near the cell equator? How does a cell robustly turn on cyclin B degradation after, and only after, the last kinetochore-spindle attachment forms? What physical mechanisms ensure both the sensitivity and robustness of metaphase/anaphase transition in the presence of noise? To address these questions, we establish a transport-reaction model that describes the intriguing spatiotemporal patterns of the mitotic players. The model is based on well-known properties of mitotic apparatus components, including kinetochores, the spindle and spindle poles. Initially, we construct a transport-only model, focusing on spatiotemporal regulation of SAC in accordance to the status of kinetochore-spindle attachments. Model results reveal nonlinear changes in the accumulation of SAC components at spindle poles; notably, this nonlinear change at the poles marks the last kinetochore-spindle attachment as greatly different from all previous attachments. With this robust spindle pole signal, we next establish a complete, transport-reaction model that includes the transport scheme and a core biochemical pathway comprising SAC proteins, cyclin B and APC/C. Our complete model demonstrates that a signal from the spindle poles could drive robust SAC silencing after and only after the last kinetochore-spindle attachment. Transport-only model Initially, we investigated the spatiotemporal redistribution of SAC components that resulted from the poleward transport that followed each proper kinetochore-spindle attachment ( Fig. 1a ). To depict the simplest scenario while retaining the biological essence, the transport-only model incorporated a single entity, called ‘cargo’. Describing SAC by a single cargo entity was a model simplification; it is a generic representative of individual SAC components that reflected their common spatial pattern. The model simulation began at a mitotic stage with a fully formed, bipolar spindle and a mixture of unattached and attached kinetochores. For this model, the key assumptions regarding transport processes were based on previous observations and are listed below. Mathematical formulations are provided in Methods. 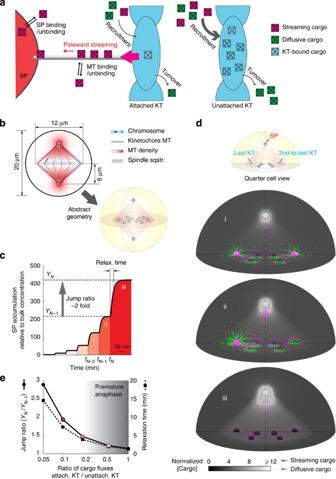Figure 1: Transport model predicts a marked spindle pole accumulation on the last kinetochore-spindle attachment. KT, kinetochore; SP, spindle pole; MT, microtubule. (a) Transport mechanism as described in the model setup. (b) Geometric setup. Upper: spatial dimensions of the cell. A sequestration (sqstr.) potential (light purple stripe) is imposed at the bipolar spindle boundary to accumulate poleward-streaming cargos to the inside of the spindle. The effects of microtubules are represented by a density field that intensifies towards spindle poles. Lower: chromosomes and kinetochores are simplified as spherical, effective kinetochore regions. Ten kinetochores are arranged at the cell equator. (c) Computed spindle pole accumulation of cargos (black solid line) with successive kinetochore-spindle attachments (dashed lines). Cargo concentration is normalized against the initial uniform concentration in the cell. The dynamics of cargo accumulation at the spindle pole are characterized by the jump ratio (YN/YN−1) and the relaxation (Relax.) time. (d) Snapshots of simulated fluxes of cargos when 2, 1 or 0 kinetochores remain unattached (labels i, ii and iii corresponding to those inc, also seeSupplementary Movie 1). The uppermost diagram illustrates reduced, quarter-cell geometry on which the fluxes are plotted for clarity. Green and magenta arrowheads: cargo fluxes. Grey scale: cargo concentration relative to the initial uniform concentration. In i and ii, most of the poleward flux from attached (attach.) kinetochores is diverted by unattached (unattach.) kinetochores and returns to the cytoplasm. In iii, poleward flux is no longer diverted; consequently, cargo rapidly and markedly accumulates on the spindle and spindle pole. (e) Signal robustness and promptness depends on reduction of cargo flux through a kinetochore on kinetochore-spindle attachment. Definitions for jump ratio and relaxation time are illustrated inc. Note that cargo flux through an unattached kinetochore is limited by the maximum capacity of a kinetochore to hold cargo proteins (due to high recruitment and low turnover, seeSupplementary Table 1), while the flux through an attached kinetochore is limited by relatively low recruitment rates. Colour-coded dots mark the parameters used in the results shown inFig. 3c. Values for model parameters and reasons for choosing those values are provided in Supplementary Table 1 and Supplementary Note 1 . Figure 1: Transport model predicts a marked spindle pole accumulation on the last kinetochore-spindle attachment. KT, kinetochore; SP, spindle pole; MT, microtubule. ( a ) Transport mechanism as described in the model setup. ( b ) Geometric setup. Upper: spatial dimensions of the cell. A sequestration (sqstr.) potential (light purple stripe) is imposed at the bipolar spindle boundary to accumulate poleward-streaming cargos to the inside of the spindle. The effects of microtubules are represented by a density field that intensifies towards spindle poles. Lower: chromosomes and kinetochores are simplified as spherical, effective kinetochore regions. Ten kinetochores are arranged at the cell equator. ( c ) Computed spindle pole accumulation of cargos (black solid line) with successive kinetochore-spindle attachments (dashed lines). Cargo concentration is normalized against the initial uniform concentration in the cell. The dynamics of cargo accumulation at the spindle pole are characterized by the jump ratio ( Y N / Y N −1 ) and the relaxation (Relax.) time. ( d ) Snapshots of simulated fluxes of cargos when 2, 1 or 0 kinetochores remain unattached (labels i, ii and iii corresponding to those in c , also see Supplementary Movie 1 ). The uppermost diagram illustrates reduced, quarter-cell geometry on which the fluxes are plotted for clarity. Green and magenta arrowheads: cargo fluxes. Grey scale: cargo concentration relative to the initial uniform concentration. In i and ii, most of the poleward flux from attached (attach.) kinetochores is diverted by unattached (unattach.) kinetochores and returns to the cytoplasm. In iii, poleward flux is no longer diverted; consequently, cargo rapidly and markedly accumulates on the spindle and spindle pole. ( e ) Signal robustness and promptness depends on reduction of cargo flux through a kinetochore on kinetochore-spindle attachment. Definitions for jump ratio and relaxation time are illustrated in c . Note that cargo flux through an unattached kinetochore is limited by the maximum capacity of a kinetochore to hold cargo proteins (due to high recruitment and low turnover, see Supplementary Table 1 ), while the flux through an attached kinetochore is limited by relatively low recruitment rates. Colour-coded dots mark the parameters used in the results shown in Fig. 3c . Full size image 1. Individual cargo underwent convection and diffusion in the cell. Each isolated cargo diffused randomly until associating with active dynein. The dynein-bound cargos began travelling poleward along microtubules towards the associated spindle pole until falling off the associated microtubule. Any dynein-bound cargo briefly diffused until binding to another microtubule and resuming poleward travel. Due to high microtubule density within the spindle and to dynein-microtubule-binding affinity, the bipolar spindle defined a compartment that concentrated active dynein-bound cargos [48] , [49] . To capture the convection–diffusion of cargos, we treated the whole cell as a spatially varying microtubule density field and incorporated both astral and spindle microtubules. Microtubule dynamics were lumped into the binding/unbinding rates of dynein-bound cargos in the microtubule density field. This consolidation is reasonable because the relevant timescale for the transported proteins to accumulate at the spindle pole (greater than minutes, as will be shown below) is much longer than the timescale for the microtubule dynamics. 2. Unattached kinetochores have very high binding affinity for individual cargo and, hence, strongly recruit them [30] , [31] , [32] , [33] , [34] , [50] , [51] . After a residence time at an unattached kinetochore, cargo returned into the cytoplasm [13] , [15] , [16] . This recruitment and release constituted constant cargo flux and exchange between any unattached kinetochore and the cytoplasm. 3. On proper spindle attachment, recruitment of cargo onto the attached kinetochore decreased because kinetochore tension caused decreases in the local effects of mitotic kinases, such as Aurora B and Plk1 (refs 52 , 53 , 54 ). For instance, Aurora B resides at the inner centromere region of mitotic chromosomes and issues the most upstream signal for recruitment of SAC components (‘cargos’) [55] , [56] , [57] , [58] , [59] ; notably, properly attached kinetochores are stretched away from the Aurora B-enriched inner centromere by spindle-generated tension [57] , [58] , [60] . In our model, the consequent reduction in the effects of mitotic kinases attenuated cargo recruitment. 4. To accurately model the finding that poleward streaming of cargos emanates only from attached kinetochores [11] , we assumed that attached and unattached kinetochores mediated opposing interconversions of cargo states. Specifically, cargos released from an unattached kinetochore diffused and were incapable of poleward streaming; only cargos from attached kinetochores underwent poleward streaming. Cargo probably underwent state changes only on kinetochores; if cargo changed state regularly in the cytoplasm, poleward streaming would rapidly diminish towards spindle poles; in addition, streaming could emerge even in the absence of attached kinetochores ( Supplementary Fig. 1 ); such possibilities contradict experimental observations [37] , [39] , [40] . Experimentally observed tension-mediated phosphoregulation of kinetochore-localized dynein and dynactin could mediate these distinctive effects on cargo by attached versus unattached kinetochores [38] . 5. Dynein-bound cargo constantly bound and released microtubules; therefore, some poleward streaming cargos reached the spindle poles while some fell off the spindle before reaching a pole. Cargos that reached a spindle pole would eventually return to the cytoplasm [11] , [13] , [15] , [16] , [36] , [39] , recycling towards the kinetochores via diffusion. In this initial model, the mitotic apparatus was represented as an interesting transport system. The kinetochore and the spindle pole functioned as terminals; dynein molecules functioned as vehicles that moved cargo. Proper kinetochore-spindle attachments connected these terminals via microtubule tracks and caused loading and movement of the vehicles; without proper attachment, cargos from unattached kinetochore diffused and were not ready for shipping. The last kinetochore attachment yields a marked polar signal This transport-only model simulated redistribution of cargos on successive kinetochore-spindle attachments in a geometrically realistic setting that mimicked a mitotic cell with a high density of microtubules within a bipolar spindle compartment ( Fig. 1b ). The model results recapitulated experimentally observed redistribution of cargos from kinetochores to the spindle pole on kinetochore-spindle attachment [11] , [31] , [36] : the model results showed that, as each additional kinetochores became properly attached to the spindle, spindle poles accumulated more cargos ( Fig. 1c ); simultaneously, the amount of cargos at attached kinetochores lessened, and the amount at unattached kinetochores remained roughly unchanged ( Supplementary Fig. 2 ). More importantly, the model predicted an emergent phenomenon; on the last kinetochore-spindle attachment, there was a marked increase in accumulation of cargos at the spindle poles; this increase constituted more than half of the final accumulation ( Fig. 1c ). We next sought to understand the uniqueness of the last kinetochore-spindle attachment. The model indicated that different kinetochore types (attached versus unattached) drove individual cargos into distinct states. Attached kinetochores equipped cargos for poleward streaming; conversely, unattached kinetochores reverted cargos to the diffusive state. These differential effects caused unattached kinetochores to divert poleward streams (see below). Snapshots taken from simulations ( Fig. 1d , also see Supplementary Movie 1 ) showed that potentially streaming cargos, which could travel poleward, were instead largely recruited to unattached kinetochores. Many streaming cargos fell off microtubules while on route to a pole, and some of these stray cargos diffused towards kinetochores. Unattached kinetochores recruited stray cargos more strongly than did attached kinetochores. Consequently, most stray cargos were recruited to unattached kinetochores; there, stray cargos reverted to the diffusive state, entered the cytoplasm and became temporarily incapable of poleward streaming. Therefore, unattached kinetochores outcompeted attached kinetochores for stray cargos and diverted poleward streaming. Notably, this diversion was mediated by cargo flux through unattached kinetochores. Any kinetochore itself could not retain cargo level above saturation; therefore, cargo levels at unattached kinetochores were saturated and essentially constant during this process ( Supplementary Fig. 2 ). After the final kinetochore-spindle attachment, all kinetochores served as open terminals that funneled all cargos throughout the entire cell into poleward streaming. Unchallenged poleward streaming then resulted in a marked increase in spindle pole accumulation. Moreover, cargo accumulation throughout the bipolar spindle compartment drastically increased while cargo levels outside the spindle dropped ( Fig. 1d , bottom). Such dynamic redistribution predicted from our model was consistent with experimental observations that green fluorescent protein-labelled Spindly, Rod and dyneins decorate the spindle and spindle pole more prominently at metaphase than during prometaphase [35] , [38] , [42] . Importantly, similar spatiotemporal patterns of the key mitotic regulators, for example, SAC proteins and cyclin B, were predictions from our model that await future experimental testing. The key contributor to the marked increase in cargo accumulation at spindle poles on the final kinetochore-spindle attachment was the absence of cargo diversion by unattached kinetochores. However, without strong recruiting power, a single unattached kinetochore could not significantly divert poleward fluxes emanating from multiple attached kinetochores. As expected, decreases in the ratio of recruitment rates between the unattached and attached kinetochores diminished the ratio between the steady-state spindle pole accumulation after and before the last kinetochore-spindle attachment ( Fig. 1e ). Furthermore, our model showed that one unattached kinetochore anywhere within the spindle compartment could divert poleward cargo streaming and keep spindle pole cargo accumulation in check ( Supplementary Fig. 3 ). Spindle pole accumulation of cargo could potentially serve as a robust readout signal for kinetochore-spindle attachments. The ratio between steady-state spindle pole accumulation after and before the last kinetochore-spindle attachment (that is, the jump ratio defined in Fig. 1c ) represented a measure of robustness of the signal for the last kinetochore-spindle attachment; a large ratio made this signal highly distinguishable from intracellular noise. The predicted large increase in spindle pole accumulation on the last kinetochore-spindle attachment thus could generate a noise-robust signal; a cell could faithfully read this signal in the presence of noise and accurately trigger SAC silencing. Transport-reaction model of SAC silencing To further investigate the potential significance of transport-mediated spatiotemporal regulation of mitotic regulators (that is, SAC components, APC/C components and cyclin B) for fidelity of SAC silencing, we incorporated the core biochemical pathway that regulates the SAC into the transport-only model to generate our complete transport-reaction model ( Fig. 2a ; also see Methods and Supplementary Methods for details). On the basis of the observed graded response of SAC activity to the number of attached kinetochores [24] , the model included a reversible, stepwise decrease in SAC activation rate on each kinetochore-spindle attachment. Importantly, the essential insight obtained from our transport-reaction model only hinged on the topology of the reaction network and was largely independent of the details of SAC biochemistry. Accordingly, the transport-reaction model incorporated only the following two additional assumptions. 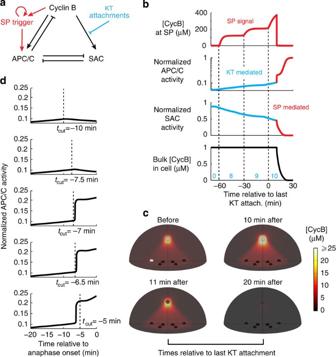Figure 2: Robust and prompt SAC silencing arises in transport-reaction model simulations. KT, kinetochore; SP, spindle pole. (a) Biochemical pathway. APC/C and SAC mutually inhibit each other. Cyclin B activates both SAC and APC/C. APC/C degrades cyclin B. Over-threshold cyclin B concentrations activate APC/C through the self-activation loop of the trigger factor. (b) Average concentrations/activity of the mitotic proteins. APC/C activity is characterized by the fraction of active APC/C of all APC/C in the whole cell. Similar definition holds for SAC activity. Cyclin B level at the spindle pole serves as the signal for the spindle pole-mediated pathway (red line, top panel). Cyan lines in plots depicting APC/C activity and SAC activity show changes during kinetochore-mediated SAC inactivation; red lines in the same plots show changes triggered by the spindle pole-issued signal after the last kinetochore attachment (attach.). Numbers of attached kinetochores at each stage of the dynamics are indicated in cyan in the bottom panel. (c) Snapshots of cyclin B distribution in the cell (also seeSupplementary Movie 2) shown on the reduced geometry. The last kinetochore-spindle attachment causes marked increase in cyclin B on the spindle and spindle pole. About 11 min later, cyclin B degradation initiates from the spindle pole. (d) Perturbation of kinetochore-spindle attachment reverses APC/C activation up to ~7 min before anaphase onset. One kinetochore is artificially ‘detached’ in the model at each specified time point (dashed lines) after all kinetochores attach properly. Figure 2: Robust and prompt SAC silencing arises in transport-reaction model simulations. KT, kinetochore; SP, spindle pole. ( a ) Biochemical pathway. APC/C and SAC mutually inhibit each other. Cyclin B activates both SAC and APC/C. APC/C degrades cyclin B. Over-threshold cyclin B concentrations activate APC/C through the self-activation loop of the trigger factor. ( b ) Average concentrations/activity of the mitotic proteins. APC/C activity is characterized by the fraction of active APC/C of all APC/C in the whole cell. Similar definition holds for SAC activity. Cyclin B level at the spindle pole serves as the signal for the spindle pole-mediated pathway (red line, top panel). Cyan lines in plots depicting APC/C activity and SAC activity show changes during kinetochore-mediated SAC inactivation; red lines in the same plots show changes triggered by the spindle pole-issued signal after the last kinetochore attachment (attach.). Numbers of attached kinetochores at each stage of the dynamics are indicated in cyan in the bottom panel. ( c ) Snapshots of cyclin B distribution in the cell (also see Supplementary Movie 2 ) shown on the reduced geometry. The last kinetochore-spindle attachment causes marked increase in cyclin B on the spindle and spindle pole. About 11 min later, cyclin B degradation initiates from the spindle pole. ( d ) Perturbation of kinetochore-spindle attachment reverses APC/C activation up to ~7 min before anaphase onset. One kinetochore is artificially ‘detached’ in the model at each specified time point (dashed lines) after all kinetochores attach properly. Full size image 1. Experimental findings show that on kinetochore-spindle attachments, cyclin B, APC/C and SAC proteins exhibit near-identical spatial redistribution [30] , [39] , [50] , [51] . Therefore, this model addressed the simplest scenario and the same transport dynamics were assigned to all three components on each kinetochore-spindle attachment. Here, APC/C referred to the combined effect of APC/C and its activator Cdc20 (ref. 1 ), and cyclin B reflected the effective activity of CDK1/cyclin B complexes [1] . 2. The model included the further assumption that cyclin B locally activated APC/C via a trigger factor only when cyclin B level at the spindle pole reached a threshold ( Supplementary Fig. 4 ). This scheme was consistent with the general consensus that threshold cyclin B levels are required for cyclin B degradation and mitotic exit [61] . The trigger factor likely represents the combined effects of the mitotic kinases concentrated at the spindle poles, for example, Plk1 and Aurora A; Plk1 and Aurora A form a positive feedback loop [62] , [63] that responds to cyclin B-CDK1 (ref. 64 ). We thus incorporated a generic auto-activation loop to represent this trigger factor [65] . This auto-activation loop ensured irreversibility of the trigger; once activated, APC/C remained active even after cyclin B level dropped. Spindle poles mediate irreversible SAC silencing The transport-reaction model simulations used the same geometry as did the transport-only model simulations ( Fig. 1b ). The model predicted the following spatiotemporal pattern of cyclin B degradation. The spindle and spindle pole became gradually enriched with cyclin B after the last kinetochore-spindle attachment ( Fig. 2b,c ; also see Supplementary Movie 2 , Supplementary Figs 5 and 6 for more details). The step change in cyclin B level at the spindle pole irreversibly activated the trigger factor, which in turn triggered the activation of APC/C and degradation of cyclin B at the spindle pole ( Fig. 2b ). The chemical activity of APC/C and degradation of cyclin B then propagated throughout the cytoplasm ( Fig. 2c ). Eventually, the whole cell was depleted of cyclin B. When 80% degradation of total cyclin B was used as the marker for anaphase onset in the model [10] , anaphase occurred ~15 min after the last kinetochore-spindle attachment ( Fig. 2b ), consistent with experiments [21] , [22] . Thus, the transport mechanism triggered prompt SAC silencing on the last kinetochore-spindle attachment. The spindle pole signal triggered a dramatic SAC-silencing process only after the last kinetochore attachment; in contrast, prior kinetochore attachments triggered weak, parallel and reversible SAC-silencing processes. Before the spindle pole signal emerged, APC/C activity increased gradually with individual kinetochore attachments ( Fig. 2b ) and degraded cyclin B slowly ( Supplementary Fig. 7 ). Perturbing any kinetochore-spindle attachment reversed increases of APC/C activity; this reversibility persisted until the irreversible, spindle pole-mediated pathway was triggered ( Fig. 2d ). Microtubule inhibitors can compromise the poleward transport of SAC components and hence block the spindle pole-mediated pathway. Therefore, drug-treated cells may manifest only the graded response on kinetochore attachments ( Supplementary Fig. 7 ), as recent experiments showed [24] , [66] . Notably, APC/C activity in drug-treated cells is indeed much lower; securin and cyclin B degradation occurs in 10 2 –10 3 min, compared with 10–20 min in untreated cells [24] , [66] . Spindle pole-mediated pathway ensures robust SAC silencing Next we investigated how the spindle pole-mediated pathway affects the SAC silencing, in comparison with the kinetochore-centric pathway. Specifically, we tuned the spindle pole-mediated pathway in the model by varying the spindle pole cargo accumulation. With small or zero spindle pole binding, the spindle pole signal was never triggered. In such cases, the cell relied solely on shutdown of kinetochore-mediated SAC activation to achieve SAC silencing ( Fig. 3a ). The kinetochore-only SAC silencing mechanism was highly susceptible to noise from the kinetochore-issued signal ( Fig. 3b ), and thus could not ensure the observed fidelity of mitosis. The risk of premature anaphase onset diminished when SAC activation remained high after kinetochores were attached ( Fig. 3b ). Due to autocatalysis of SAC by the template mechanism [17] , [19] , a high residual level of active SAC may persist in cytoplasm even after the final kinetochore attachment. However, high residual SAC activation could hinder SAC silencing and cause mitotic arrest ( Fig. 3a ). This result is consistent with the previous theoretical work [29] . As such, the kinetochore-centric pathway alone was either (1) not robust or (2) ineffective in SAC silencing. 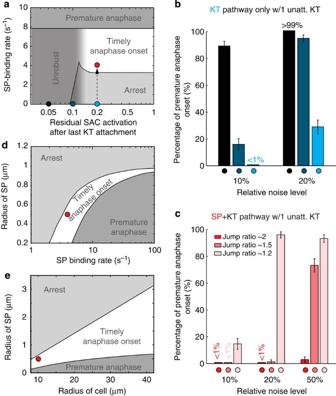Figure 3: Robust SAC silencing requires spindle pole-mediated signalling and proper spindle pole size. KT, kinetochore; SP, spindle pole. Timely anaphase onset: cyclin B degradation after the last kinetochore-spindle attachment. Premature anaphase: cyclin B degradation before the last kinetochore-spindle attachment. Arrest: insufficient cyclin B degradation. (a) Phase diagram of mitotic fate on residual SAC activation versus spindle pole-binding rate. The residual SAC activation is defined as a fraction—the SAC activation rate after all kinetochores are attached divided by the original SAC activation rate before any kinetochore is attached. The spindle pole-binding rate essentially tunes the effect of the spindle pole-mediated signalling pathway. The grey ‘unrobust’ zone covers parameter space with high risk of premature anaphase onset caused by noise as shown in panelb. (b) Percentage of all cells with only the kinetochore-centric pathway and one unattached (unattach.) kinetochore that undergo premature anaphase onset (80% cyclin B degradation) within 1 h. Colour-coded dots mark the corresponding parameters in phase diagrama. Noise was imposed on the SAC activation rate to simulate the noisy kinetochore signal (see Methods). Corresponding mean relative SAC activation rates with one unattached kinetochore for the three cases are 14.5% (dark blue), 19% (medium blue) and 28% (light blue), respectively (Supplementary Fig. 11). (c) Percentage of all cells with two pathways (kinetochore-centric and spindle pole-mediated) and one unattached kinetochore that undergo premature anaphase onset within 1 h. Noise was imposed on the effects of cyclin B signal (see Methods). Colour codes show cases with different jump ratios. Colour codes mark corresponding parameters and specific jump ratios inFig. 1e. Inb,c, 300 stochastic partial differential equation simulations were run for each parameter set. Error bars (1.96 × s.e.m.) and percentage numbers illustrate 95% confidence interval determined via the Wald method and probability calculation, respectively (see Methods). (d) Phase diagram of mitotic fate given spindle pole size and binding rate. (e) Phase diagram of mitotic fate given cell size and spindle pole size. In accordance with experimental observations67, length and diameter of spindles scale with cell size in all simulations. Figure 3: Robust SAC silencing requires spindle pole-mediated signalling and proper spindle pole size. KT, kinetochore; SP, spindle pole. Timely anaphase onset: cyclin B degradation after the last kinetochore-spindle attachment. Premature anaphase: cyclin B degradation before the last kinetochore-spindle attachment. Arrest: insufficient cyclin B degradation. ( a ) Phase diagram of mitotic fate on residual SAC activation versus spindle pole-binding rate. The residual SAC activation is defined as a fraction—the SAC activation rate after all kinetochores are attached divided by the original SAC activation rate before any kinetochore is attached. The spindle pole-binding rate essentially tunes the effect of the spindle pole-mediated signalling pathway. The grey ‘unrobust’ zone covers parameter space with high risk of premature anaphase onset caused by noise as shown in panel b . ( b ) Percentage of all cells with only the kinetochore-centric pathway and one unattached (unattach.) kinetochore that undergo premature anaphase onset (80% cyclin B degradation) within 1 h. Colour-coded dots mark the corresponding parameters in phase diagram a . Noise was imposed on the SAC activation rate to simulate the noisy kinetochore signal (see Methods). Corresponding mean relative SAC activation rates with one unattached kinetochore for the three cases are 14.5% (dark blue), 19% (medium blue) and 28% (light blue), respectively ( Supplementary Fig. 11 ). ( c ) Percentage of all cells with two pathways (kinetochore-centric and spindle pole-mediated) and one unattached kinetochore that undergo premature anaphase onset within 1 h. Noise was imposed on the effects of cyclin B signal (see Methods). Colour codes show cases with different jump ratios. Colour codes mark corresponding parameters and specific jump ratios in Fig. 1e . In b , c , 300 stochastic partial differential equation simulations were run for each parameter set. Error bars (1.96 × s.e.m.) and percentage numbers illustrate 95% confidence interval determined via the Wald method and probability calculation, respectively (see Methods). ( d ) Phase diagram of mitotic fate given spindle pole size and binding rate. ( e ) Phase diagram of mitotic fate given cell size and spindle pole size. In accordance with experimental observations [67] , length and diameter of spindles scale with cell size in all simulations. Full size image The spindle pole-mediated pathway resolved the dilemma between robustness and effectiveness for SAC silencing ( Fig. 3a ). The spindle pole signal triggered SAC silencing via a separate pathway at a distinct location; with this trigger, SAC activation could remain high and buffer against noise while awaiting the spindle pole signal for irreversible silencing ( Fig. 3a , dashed arrow). The spindle pole pathway itself was highly robust even with noise because of the tremendous signal increase on the last kinetochore attachment. This pathway could buffer against noise up to 50% of the signal level ( Fig. 3c , columns marked by bright red dots). The spindle pole-mediated SAC-silencing pathway could resolve the robustness problem intrinsic to the gradual loss of SAC activation via the kinetochore pathway. Thus, by taking into account the observed spatiotemporal pattern of key mitotic regulators during prometaphase and metaphase, our model predicted an emergent phenomenon. Unattached kinetochores diverted key mitotic regulators from poleward streaming, and thereby prevented them from entering spindle poles; this diversion abated when the last kinetochore became attached. With unchallenged poleward streaming, there was a large increase in spindle pole accumulation of key mitotic regulators. This large signal increase dictated robust and prompt SAC silencing after, and only after, the last kinetochore-spindle attachment. Such behaviour was evident over a wide range of model parameters ( Supplementary Fig. 8 ). The model thus established a coherent picture that put the complex spatiotemporal patterns of key mitotic regulators into perspective. In particular, the model indicated a functional role for transporting mitotic proteins between the kinetochores, spindle and spindle poles during mitosis. The drastic reduction in cargo recruitment rate onto a kinetochore on kinetochore-spindle attachment was critical for both robustness and promptness of SAC silencing ( Fig. 1e ). In particular, reduced differences in recruitment rates between unattached and attached kinetochores abrogated signal robustness and increased risk of premature SAC silencing (columns marked by lighter red dots in Fig. 3c , also the grey region in Fig. 1e ). On the other hand, minimal cargo recruitment onto attached kinetochores restricted total poleward flux from kinetochores and delayed the accumulation of a threshold signal at the spindle pole (dashed line in Fig. 1e ). Therefore, proper regulation of recruitment rates at attached kinetochore was important for both robustness and promptness of anaphase onset. Robust SAC silencing requires proper spindle pole size In our model, the spindle pole effectively served as a counting apparatus that counted signals from each attached kinetochore; the mitotic cell used this apparatus to determine when to silence SAC and degrade cyclin B. Our model predicted that for a given spindle pole size, only intermediate cargo-binding rates at the spindle pole could tightly couple timing of SAC silencing with the last kinetochore-spindle attachment ( Fig. 3d ). Low binding rates prevented spindle poles from accumulating enough cyclin B to trigger SAC silencing; the cell was then arrested in mitosis, even when each kinetochore was properly attached to the spindle. Conversely, high binding rates allowed spindle poles to accumulate the threshold level of cyclin B before the last kinetochore-spindle attachment; therefore, high rates resulted in premature SAC silencing and premature anaphase onset. Similarly, spindle pole size also affected the concentration of key mitotic players at the spindle poles ( Supplementary Fig. 8h ). Small spindle poles resulted in (1) poleward fluxes that streamed into small spaces and (2) high concentrations of SAC cargos at spindle poles; cyclin B levels easily rose above threshold levels and triggered premature SAC silencing. Conversely, large spindle poles (1) resulted in dilute polar concentrations of cyclin B, (2) prevented accumulation of threshold levels of cyclin B and (3) caused aberrant mitotic arrest. These findings indicated that size mattered. Notably, the model further predicted that spindle pole size and cell size needed to be properly correlated to support timely anaphase onset ( Fig. 3e ). Large cells contain larger amounts of mitotic regulators. Consequently, dynein-mediated poleward transport conveyed stronger streams of proteins towards the spindle pole. If spindle pole size remained constant as cell sizes varied, then in large cells, cyclin B would overaccumulate at the spindle pole and cause premature SAC silencing. However, in large cells, large spindle pole sizes would dilute protein concentrations at spindle poles and lead to correct timing for SAC silencing. Conversely, smaller cells needed smaller spindle poles to avoid untimely mitotic arrest. This model result thus offered a possible explanation for the observed correlation between spindle pole size and cell size in mouse embryos in the first few mitoses [67] . Our model provided a mechanism that could underlie a critical function role of the spatiotemporal dynamics of mitotic regulators in SAC silencing. The entire mitotic apparatus in the model was conceived of as a coherent transport system comprising kinetochores, a bipolar spindle and spindle poles. Model simulations demonstrated that spatiotemporal regulation of mitotic regulators mediated by this transport system ensured robust SAC silencing after, and only after, all kinetochores became properly attached ( Fig. 4 ). Specifically, proper kinetochore-spindle attachment resulted in dynein-mediated poleward flux and spindle pole accumulation of key mitotic regulators (SAC proteins, cyclin B and APC/C). This flux was diverted by any unattached kinetochore because unattached kinetochores exhibited stronger recruitment of mitotic players than did attached kinetochores. Strong antagonism between unattached kinetochores and attached kinetochores significantly restrained spindle pole accumulation. When all kinetochores became properly attached, poleward flux was unchallenged; the unchallenged flux resulted in a marked increase in spindle pole accumulation, more than the combined accumulation caused by all previous kinetochore-spindle attachments. This nonlinearity in spindle pole accumulation conferred a robust signal that triggered SAC silencing after, and only after, the last kinetochore-spindle attachment. Subsequently, SAC silencing propagated from the spindle poles throughout the cell ( Figs 2c and 4 ). 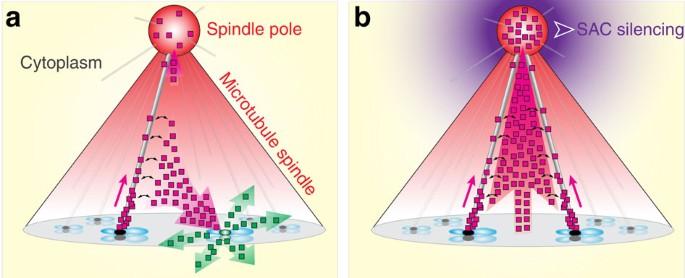Figure 4: Model summary. Our transport-reaction model indicated that robust SAC-silencing signal after and only after the last kinetochore-spindle attachment arises from spatial regulation of mitotic proteins. (a) Streaming mitotic proteins (red square) emanate from the attached kinetochores (black oval), but the poleward flux is strongly diverted by any unattached kinetochore (green oval), where the streaming proteins revert to the diffusive state (green square). (b) When all the kinetochores properly attach to the spindle, strong, undiverted poleward fluxes cause significant protein accumulation at the spindle pole, and generate a robust signal that triggers SAC silencing. This trigger propagates from the spindle pole throughout the cell. For clarity, fluxes of mitotic proteins are only shown for the two kinetochores in the foreground. Distribution of the squares does not reflect spatial distribution of mitotic proteins. Translucent magenta arrows: fluxes of streaming proteins. Translucent green arrows: fluxes of diffusive proteins. Solid magenta arrows: streaming proteins along the microtubules. Black arrows: binding/unbinding of streaming proteins with microtubules. Figure 4: Model summary. Our transport-reaction model indicated that robust SAC-silencing signal after and only after the last kinetochore-spindle attachment arises from spatial regulation of mitotic proteins. ( a ) Streaming mitotic proteins (red square) emanate from the attached kinetochores (black oval), but the poleward flux is strongly diverted by any unattached kinetochore (green oval), where the streaming proteins revert to the diffusive state (green square). ( b ) When all the kinetochores properly attach to the spindle, strong, undiverted poleward fluxes cause significant protein accumulation at the spindle pole, and generate a robust signal that triggers SAC silencing. This trigger propagates from the spindle pole throughout the cell. For clarity, fluxes of mitotic proteins are only shown for the two kinetochores in the foreground. Distribution of the squares does not reflect spatial distribution of mitotic proteins. Translucent magenta arrows: fluxes of streaming proteins. Translucent green arrows: fluxes of diffusive proteins. Solid magenta arrows: streaming proteins along the microtubules. Black arrows: binding/unbinding of streaming proteins with microtubules. Full size image The key difference between our model and previous models was treating the whole spindle structure as signal mediator for SAC. All previous models for SAC [23] , [27] , [28] , [29] regard kinetochores as the only loci that mediate SAC activation and SAC silencing; consequently, previous models ignore the spatiotemporal regulation of SAC activity. Cells can house a large number of kinetochores (10 1 –10 3 ), these models inevitably face the robustness problem; specifically, final kinetochore-spindle attachment could not reliably produce a robust signal distinct from those of previous kinetochore attachments. In the most recent SAC-silencing model by He et al . [23] , if the input signal faces 10 or 20% relative noise, the rates of premature cyclin B degradation are high as 14 and 55%, respectively ( Supplementary Fig. 9 ), whereas our model was almost error free under the same conditions ( Fig. 3c ). In our model, poleward transport translated the number of attached kinetochores into a nonlinear signal from the spindle pole; this signal robustly marked the last kinetochore-spindle attachment. Our model indicated that different parts of the mitotic apparatus each had distinct functional roles in SAC signalling. Kinetochores generated information by changing cargo states; the spindle conveyed the information as poleward transport streams; spindle poles integrated the information and generated a nonlinear signal readout. Our model further indicated distinct behaviours and differential functional roles of two coexisting SAC-silencing pathways—a kinetochore-mediated and a spindle pole-mediated pathway. Gradual loss of kinetochore-mediated SAC activation on kinetochore attachments generated low-level, reversible APC/C activation. This low-level APC/C activation may clear early mitotic regulators that are more sensitive to APC/C and prime the cell for further mitotic progression. The spindle pole signal was robust against noise and launched the final SAC silencing and irreversible transition into anaphase. The coexistence of these two pathways could generate reversible SAC silencing that persisted until minutes before anaphase onset ( Fig. 2d ). The spatial component of the regulation in our model reconciled a long-standing dilemma between promptness of SAC silencing and the potency of SAC activity from a single unattached kinetochore. A previous seminal study [29] indicates that potent SAC activity requires that SAC deactivation is slower than SAC activation. Yet, the small size of kinetochores physically limits the pace of SAC activation [68] . Although a Mad2 template mechanism can amplify SAC activation in cytoplasm, the amplified activation rate remains meagre [19] , and the corresponding SAC silencing is slow, >10 2 min (ref. 19 ). To achieve rapid SAC silencing after the last kinetochore becomes attached, each previous model overstretches the SAC activation pace so that it can outcompete SAC deactivation [23] , [27] , [28] , [29] , [68] . For example, the model by Sear and Howard [28] pushes the SAC activation rate to three orders of magnitude larger than experimental measurements (~6 μM −1 s −1 assumed versus 0.003 μM −1 s −1 measured [19] ). Our model is free of this dilemma because SAC silencing was triggered through the spindle pole pathway that was spatially separated from kinetochores. Thus, the pace of SAC silencing was essentially decoupled from the quenching of SAC activation after kinetochore attachment ( Supplementary Fig. 10 ). The model in its present form only captured the most salient features of SAC silencing. Future experimental findings can help improve the model with more realistic details, including the feedback of cyclin B level onto kinetochore dynamics as mentioned above. Furthermore, ample evidence indicates that kinase environments differ between attached and unattached kinetochores [54] , [60] ; however, our current model used only a phenomenological switch of parameters to represent the differential effects of these different kinetochore types on poleward streaming. A more realistic model requires future experiments that resolve the detailed phosphoregulation pathway of dynein/cargo dynamics. In addition, the SAC comprises multiple components that may not all travel together; they might dissociate from and rebind with each other over time. The current model simulated only average SAC activity, and thus imparted the same transport dynamics to all SAC components. Future efforts will explore the effects of disparate transport dynamics of SAC components on the SAC-silencing process. Last, the threshold spindle pole signal level for activating the trigger factor profoundly affects the fate of mitosis in our model. While a particular threshold value was certainly assumed for our model, robust and efficient SAC silencing was supported by a reasonably broad range (250–450 μM) of threshold values ( Supplementary Fig. 4 ; Supplementary Methods ). This model result actually reflected another facet of the phase diagrams shown in Fig. 3a,d,e —SAC silencing was ultimately determined by spindle pole accumulation relative to a threshold value. This conclusion led to an interesting question: how did the cell determine the spindle pole threshold signal? We do not have an answer, but we will use future experimental findings to develop more hypotheses. In sum, we modelled the mitotic apparatus as a transport system that operates in accordance with the status of kinetochore-spindle attachments. A coherent picture emerged from our model: the spindle pole integrated information from individual kinetochore to generate a mitotic signal. The highly nonlinear nature of this signal ensured robust SAC silencing after, and only after, all kinetochore-spindle attachments formed properly. This model thus provided a unique solution to the robustness problem of SAC silencing in mitosis. It underscored the functional role of spatiotemporal regulation of SAC activity and established a conceptual framework for understanding the mechanism that controls fidelity of mitosis. Models The qualitative essences of the ‘Transport-only Model’ and those of ‘Transport-Reaction Model’ were translated into compartmentalized partial differential equations. These compartmentalized equations described the distinct spatiotemporal dynamics and biochemical regulatory events at kinetochores and spindle poles and in the cytoplasm. Both models shared the same geometric model setup. Each model cell was divided into N KT +1 compartments that included the cytoplasm and N KT kinetochores ( Fig. 1b ). In addition, the spindle pole was defined as a virtual domain in the mathematical sense. In each model, a bipolar microtubule density field with density increases towards spindle poles was used to implicitly describe the effects of a bipolar spindle. This microtubule density field determined binding rates between poleward streaming cargos and microtubules. In addition, this microtubule density field defined a potential that promoted accumulation of streaming cargos to the inside of the bipolar spindle (see Supplementary Note 1 for details). Below, detailed equations are presented for the transport-only model and transport-reaction model. COMSOL Multiphysics 4.3 was used to solve the partial differential equations and for all stochastic simulations; MATLAB was used to process all generated data. Transport-only model Three cargo states were used to depict the spatiotemporal dynamics of any cargo in the cytoplasm. Y 00 represented diffusive cargos, which were not capable of poleward streaming; Y 00 likely represented a cargo state without active dynein. Y 1 represented streaming, microtubule-bound cargos that were actively travelling poleward along microtubules. Y 0 represented streaming cargos temporarily unbound from any microtubule and diffusing in the cytoplasm. The Y 1 ↔ Y 0 interconversion represented the binding and release between streaming cargos and microtubules. The spatiotemporal dynamics of cargos in the cytoplasm were governed by equations (1)–(3). In cytoplasm: In equations (1)–(3), D Dyn and D MT denote the diffusion coefficients of the active dynein-cargo complex in the cytoplasm and along the microtubule, respectively. D Y denotes the cytoplasmic diffusion coefficient of diffusive cargos. V denotes the velocity of streaming cargos along a microtubule, pointing towards the nearest spindle pole, as indicated by . k onMT denotes the binding rate of streaming cargos to microtubule (that is, Y 0 → Y 1 ), and is proportional to the microtubule density ρ MT that concentrates towards the spindle pole (see Supplementary Note 1 for detailed setup). k offMT denotes the unbinding rate of streaming cargos from the microtubule (that is, Y 1 → Y 0 ). U ext denotes the sequestration potential imposed by spindle on any streaming cargos (see Supplementary Note 1 for details). k B denotes the Boltzmann constant, and T denotes temperature. To capture the integration of poleward fluxes at spindle poles, the spindle pole area was assigned an additional cargo state, Y P ; Y P represented cargos sequestered at a spindle pole. To model sequestration and release of streaming cargos by spindle pole material, Y P could interconvert with streaming cargos ( Y 1 or Y 0 ) inside the spindle pole domain. The spatiotemporal dynamics of cargos inside the spindle pole were governed by equations (4)–(7). At spindle poles: In equations (4)–(7), k onSP and k offSP denote the binding and unbinding rates of cargos to and from the spindle pole, respectively. The diffusion coefficient of the spindle pole-sequestered cargo, D P , was set to equal D Dyn . Within the spindle pole domain, and are the chosen rates for binding and release, respectively, between cargos and microtubules. With these parameter choices, equations (4)–(7) essentially characterized the integration of the poleward streams at the spindle pole with the following simple process. When cargos entered the spindle pole, they fell off microtubules instantaneously, and bound spindle pole material with a certain residence time. When unbound to either spindle pole material or microtubules, cargos could freely diffuse out of the spindle pole domain. The overall effect of the spindle pole dynamics was partial sequestration of cargos arriving at the spindle pole. Qualitatively, this effect did not rely on the detailed assumptions of the spatial dynamics of cargos within the spindle pole area. Kinetochores were the key loci for interconversion between streaming ( Y 1 , Y 0 ) and diffusive ( Y 00 ) cargos. To realize such interconversion, we assumed the following process at kinetochores. First, kinetochores recruited cargos, regardless of cargo state. Once entering a kinetochore domain, a cargo was designated by a new, kinetochore-bound state; Y K n denotes this state, where n labels the n th kinetochore. On release from a kinetochore domain, the cargo state depended on the attachment state of the kinetochore: unattached kinetochores released only diffusive cargos, and attached kinetochores released mostly streaming cargos. This spatiotemporal dynamics was governed by equation (8), with boundary fluxes defined in equations (9)–(16), , , , , . At the n th kinetochore: where the diffusion coefficient D K = D Dyn . Flux across boundary of unattached kinetochore: Flux across boundary of attached kinetochore: In equations (9)–(16), , , , , , n refers to the unit normal vector of the kinetochore boundary. Γ ’s with corresponding subscripts denote the fluxes of cargos across the kinetochore boundary. k onKTu and k onKTt denote recruitment rates of cargos onto unattached and attached kinetochores, respectively. The term sets the saturating limit of kinetochore-bound cargos. k offKT denotes the turnover rate of diffusive cargos into the cytoplasm. k DoffKT denotes the release rate of streaming cargos from an attached kinetochore onto kinetochore microtubules. Note that each attached kinetochore kept releasing diffusive cargos. But since this release rate was much smaller than that for streaming cargos ( Supplementary Table 1 ), the efflux of diffusive cargos from an attached kinetochore was negligible. This term was kept for consistency of the physical picture: if not assembled with dynein and activated for poleward transport, the cargo would nevertheless turn over spontaneously from a kinetochore. Each kinetochore-spindle attachment caused a reduction in the recruitment rate, from k onKTu to the smaller k onKTt , and launch of k DoffKT at the kinetochore. We assumed that recruitment was more sensitive to kinetochore attachment than the activation of dynein-mediated poleward transport. To characterize the gradual stabilization of kinetochore-spindle attachment [69] , we imposed a 5-min delay between the reduction of k onKT and the launch of k DoffKT . Parameter values for equations (1)–(16), , , , , ,  and the rationales for the parameter choices are listed in Supplementary Table 1 and Supplementary Note 1 . Transport-reaction model The full transport-reaction model combined the transport dynamics described above with known biochemical reactions in the SAC pathway. The major biochemical species from the SAC pathway that were defined as cargo in this model were SAC ( M ), APC/C ( A ), cyclin B ( C ) and a spindle pole trigger factor ( X ; Fig. 2a ). In contrast to other species, the trigger factor X did not bind microtubules and hence did not undergo convection. X adopted only the diffusive state in the cytoplasm. Spatial regulation of X included only interconversion between cytoplasmic diffusion and binding at the spindle poles. We provide the complete set of equations for X at the end of this section. The transport-reaction equations for SAC, APC/C and cyclin B took the general form of equations (17)–(21), , , , . In addition to the biochemical reactions, SAC, APC/C and cyclin B were assumed to undergo the same transport process as defined for the cargo Y in the transport-only model. Accordingly, the spatial regulation terms in equations (17)–(21), , , ,  were the same as those in the transport model for different compartmental domains (equations (1)–(8)). As the biochemical reactions were modelled as volumetric for each compartment, they were not added to the equations for the flux across compartment boundaries. In equations (17)–(21), , , , , superscripts i and a indicate chemically inactive and active forms, respectively. Since cyclin B dynamics were controlled by degradation, cyclin B took only the active form. Most reaction rates are conveniently denoted by k with meaningful subscripts. For example, k dAwM denotes deactivation of A by M , and k aAwX denotes activation of A by X . Similar nomenclature rule applies to most reaction rates. The term f A = A a /( A a + A i ) denotes the local fraction of active APC/C, and is used to represent the average effectiveness of APC/C on cyclin B. The degradation of cyclin B by APC/C is characterized by a Hill function form with Hill coefficient H and half transition level K mdCwA (see Supplementary Fig. 11 ; Supplementary Note 2 for details and rationales). In particular, the kinetochore-mediated SAC activation was approximated by two terms, k aMKT and k aMCat ; the first, k aMKT , denotes the low rate that represented the direct activation of SAC at unattached kinetochores. Thus, the rate decreased stepwise on each kinetochore attachment ( Supplementary Fig. 11 ). The second, k aMCat , denotes the larger rate that reflected the essence of SAC activity amplification through the template mechanism. On each kinetochore attachment, k aMCat also decreased, but with a long relaxation time, denoted τ DaM ( Supplementary Fig. 11 ). This long relaxation time has been suggested by other theoretical works, because of the diffusive catalytic process in the template mechanism [19] , [28] , [29] . k aMCat may not have become zero after all kinetochores became attached ( Supplementary Fig. 11 ) if autocatalysis was sufficiently strong [29] . For clarity, we give an example of the complete partial differential equations for active SAC in equations (22)–(37), , , , , , . The equations for inactive SAC, active and inactive APC/C and active cyclin B were similarly constructed. The complete set of equations is given in Supplementary Methods . Active SAC included the following species: (1) active SAC undergoing poleward streaming, ; (2) active SAC capable of poleward streaming, but not bound to a microtubule, ; (3) active SAC in diffusive state, not capable of poleward streaming, ; (4) active SAC in the n th kinetochore, ; (5) spindle pole-bound active SAC, . In cytoplasm: At spindle poles: On the n th kinetochore: Flux across unattached kinetochore: Flux across attached kinetochore: Equations (29)–(37), , , , , ,  present processes that were identical to those in the transport-only model: once having crossed the kinetochore boundary, an active SAC component in cytoplasm, , , or , became a new kinetochore-bound entity, . In equations (22)–(28), two terms, and , denote local concentrations of chemically active APC/C and cyclin B, respectively, regardless of the transport state (terms in the bracket exist for spindle pole region only). The spatiotemporal dynamics and biochemical activity of X factor are described simply by equations (38)–(49), , , , , , , , , , , where GK refers to the Goldbeter–Koshland function, a commonly used function to describe auto-activation [65] . In cytoplasm: At spindle poles: On the n th kinetochore: Flux across boundary of unattached or attached kinetochore: A complete list of parameter values for the transport-reaction model and the rationales for the parameter choices are provided in Supplementary Table 2 , Supplementary Table 3 and Supplementary Note 2 . Stochastic simulations for evaluation of signal robustness To evaluate the signal robustness in the transport-reaction model, we ran stochastic simulations to estimate the likelihood of noise-induced premature anaphase onset when just one unattached kinetochore persisted in a cell. In a single simulation, premature anaphase onset registered only if cyclin B level dropped to below 20% of its maximal value within 1 h. For the kinetochore-only pathway, we focused on the robustness of the kinetochore-mediated SAC inactivation, that is, reduction of SAC activation with each kinetochore attachment. Therefore, we imposed stochastic noise on the global effective SAC activation rate. For the spindle pole pathway, we focused on noise robustness against fluctuations in the spindle pole signal, that is, cyclin B activity. Noise in cyclin B signal included fluctuations in cyclin B concentration and biochemical activity. A high cyclin B concentration at the spindle pole led to very small concentration fluctuations. With ~100 nM bulk concentration for most SAC components ( Supplementary Table 2 ), any spindle pole with ~0.5 μm 3 volume and a cargo concentration several hundred times the bulk concentration accumulated at least 10 4 molecules of each biochemical species. The relative fluctuations in concentration were thus on the order of 1%. The fluctuations in biochemical activities, on the other hand, could reach higher levels, stemming from conformational fluctuations, variations in protein expression level and so on. Here we simply lumped these stochastic effects into dynamic noise in the biochemical reaction rates of processes mediated by cyclin B. Kinetochor e-only pathway . Noise was imposed on the activation rate of SAC, whereas reactions involving APC/C, cyclin B or the trigger factor were modelled as noiseless. Furthermore, to single out the stochastic effect of the kinetochore-only pathway, in these simulations we excluded any spindle-mediated spatial regulation, including convection and spindle pole accumulation; consequently, the streaming cargo states were also excluded. Therefore, the equations for SAC in the cytoplasm, for instance, simply read as equations (50) and (51). The terms are excluded. and herein denote rate values corresponding to the stage with one unattached kinetochore ( Supplementary Fig. 11a ). The noise was scaled against , which denotes the overall SAC activation rate from all kinetochores when none are attached. The term ξ ( t ) denotes the time series of relative stochastic noise with ‹ ξ ( t )›=0 and ‹ ξ 2 ( t )›= q 2 , where q is the relative noise level shown in Fig. 3b,c . Construction of ξ ( t ) is elaborated in Supplementary Methods . The fluxes across the kinetochores took the same form as equations (33) and (37). The complete set of equations for stochastic simulation of kinetochore-centric pathway is given in Supplementary Methods . Spindle pole pathway . Noise was imposed on the reactions controlled by cyclin B. To single out the effect of noise in the spindle pole signal, we ignored any noise outside the spindle pole. The chemical reaction terms at the spindle pole were thus modified to equations (52)–(58), , , , , , , whereas the reaction terms outside the spindle pole remained unchanged. Here, the noise ξ ( t ) was constructed in the same way as described above. The complete transport-reaction equations at the spindle pole and detailed stochastic simulation scheme are given in Supplementary Methods and in Supplementary Fig. 12 . Choice of sample size and statistics . The rate of chromosome mis-segregation is estimated to be about 1 per 100 divisions in normal diploid cells [70] . To characterize such a small probability, particularly in the nominal case, we chose to run 300 independent stochastic simulations for each case. If no premature anaphase onset was identified in all 300 simulations, then the true probability of premature anaphase onset is <1% with 95% confidence. This is because probability ( P <0.01|no event out of N samples)=1–(1–0.01) N +1 and thus 95% confidence requires sample size N >297. By symmetry, if all 300 simulations gave rise to premature anaphase onset, then the probability of premature anaphase onset is >99% with 95% confidence. For cases with premature anaphase onsets numbered between 1 and 299, we used the Wald method to estimate the 95% confidence interval for the probability of premature anaphase onset, that is, , where is the observed frequency of premature anaphase onset and N =300 is the sample size. How to cite this article: Chen, J. and Liu, J. Spatiotemporal model for silencing of the mitotic spindle assembly checkpoint. Nat. Commun. 5:4795 doi: 10.1038/ncomms5795 (2014).